Widespread impact of horizontal gene transfer on plant colonization of land In complex multicellular eukaryotes such as animals and plants, horizontal gene transfer is commonly considered rare with very limited evolutionary significance. Here we show that horizontal gene transfer is a dynamic process occurring frequently in the early evolution of land plants. Our genome analyses of the moss Physcomitrella patens identified 57 families of nuclear genes that were acquired from prokaryotes, fungi or viruses. Many of these gene families were transferred to the ancestors of green or land plants. Available experimental evidence shows that these anciently acquired genes are involved in some essential or plant-specific activities such as xylem formation, plant defence, nitrogen recycling as well as the biosynthesis of starch, polyamines, hormones and glutathione. These findings suggest that horizontal gene transfer had a critical role in the transition of plants from aquatic to terrestrial environments. On the basis of these findings, we propose a model of horizontal gene transfer mechanism in nonvascular and seedless vascular plants. Horizontal gene transfer (HGT) is the process of genetic movement between species. Traditionally considered to be predominant in prokaryotes [1] , HGT now appears to be widespread in microbial eukaryotes [2] . As an efficient mechanism to spread evolutionary success, HGT may introduce genetic novelties to recipient organisms, thus facilitating phenotypic variation and adaptation to shifting environments or allowing access to new resources. The novelties introduced by HGT range from virulence factors in pathogens [3] , [4] , food digestive enzymes in nematodes and rumen ciliates [5] , [6] , to anaerobic metabolism in intracellular parasites [6] , [7] . Although HGT in prokaryotes and unicellular eukaryotes has been under some extensive studies and well documented [8] , [9] , [10] , how HGT has contributed to the evolution of complex multicellular eukaryotes, such as animals and plants, remains elusive. Presumably because of the barrier of germline in animals and apical meristem in plants [9] , [11] , HGT is generally believed to be rare and insignificant in complex multicellular eukaryotes, except for organisms in a symbiotic relationship [12] , [13] and for plant mitochondrial genes [14] , [15] . This belief, however, has been cast in doubt by reports of acquired genes in invertebrates and plants from free-living organisms [5] , [16] , [17] , [18] . Importantly, because all multicellular eukaryotes are derived from unicellular ancestors, this belief largely discounts the dynamic nature of HGT and the contribution of ancient HGT to the evolution of multicellular lineages [19] . Therefore, to better understand the role of HGT in eukaryotic evolution, it is critical to reassess the occurrence and biological functions of horizontally acquired genes in multicellular eukaryotes. Land plants emerged from charophycean green algae about 480–490 million years ago [20] . During their colonization of land, plants gradually evolved complex regulatory systems, body plan and phenotypic novelties that facilitated their adaptation to and radiation in terrestrial environments [21] . Because of the importance of HGT in the adaptation of organisms to new niches, we decided to investigate whether such habitat and developmental transition was aided by acquisition of novel genes, especially those during early evolution of land plants. Thus far, although the role of HGT in the evolution of land plants, especially flowering plants, has long been speculated [22] , there are very few reported cases of HGT in land plants that are related to nuclear genes [23] , [24] , [25] . We here present evidence for the widespread and significant impact of HGT of nuclear genes on plant colonization of land based on analyses of the moss Physcomitrella patens, an extant representative of early land plants. We further propose a model for gene acquisition in nonvascular and seedless vascular plants and discuss the cumulative impact of HGT on multicellular eukaryotes. HGT-derived genes in land plants Eukaryotic genomes contain many genes of prokaryotic origin, most of which are derived from mitochondria and plastids [26] . Gene transfer from these organelles to the nucleus, often called endosymbiotic gene transfer (EGT), has been studied in many eukaryotic groups [27] , [28] , [29] and will not be included here. In this study, we identified genes in land plants that were acquired independently from other sources, primarily based on phylogenomic analyses of the moss P. patens . Whenever possible, independent evidence such as restricted taxonomic distribution and uniquely shared genomic characters (for example, indels or domain structures) were also considered. To reduce the complication arising from differential gene losses, we focused on identifying genes acquired from prokaryotes and viruses. Genes acquired from fungi were also identified because of the role of mycorrhizae in land plant evolution [30] and available evidence for HGT between mycorrhizal partners [25] . Furthermore, because genes acquired by the common ancestor of Plantae (green plants, red algae and glaucophytes) have been under some detailed analyses [31] , [32] , [33] , this study only identified genes in P. patens that were acquired after the separation of green plants from red algae and glaucophytes. With the annotated protein sequences of P. patens as input, 910 genes were identified using AlienG [34] as potentially of prokaryotic, fungal or viral origin. Among these 910 genes, 394 were removed from further analyses because of their locations on short scaffolds or their high percent-identities with cyanobacterial sequences, which is often suggestive of plastid origin. Of the remaining 516 genes, 32 genes of four families had identifiable homologues only in prokaryotes or fungi; 96 genes of 53 families showed a monophyletic relationship between sequences of green plants and those from prokaryotes, fungi or viruses in phylogenetic analyses, with bootstrap support of 80% or higher from either maximum likelihood or distance analyses or both. 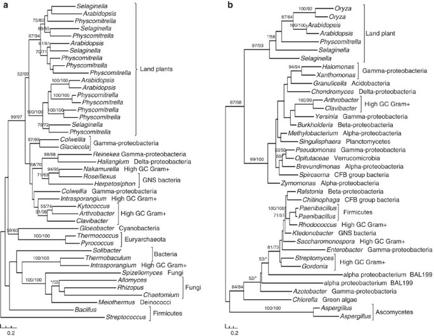Figure 1: Molecular phylogenies of subtilases (a) and vein patterning 1 (VEP1) (b). Numbers above branches show bootstrap values from maximum likelihood and distance analyses, respectively. Asterisks indicate values <50%. In total, 128 genes of 57 families were identified as derived from prokaryotes, fungi or viruses ( Table 1 ; Figs 1 and 2 ; Supplementary Information ). Twenty-four of these gene families in green plants also share unique indels and amino acid residues with their putative donors. The online Supplementary Data show the taxonomic distributions, multiple sequence alignments, molecular phylogenies and other relevant information for the 57 gene families we have identified in this study. Table 1 Horizontally acquired genes identified in Physcomitrella patens . Full size table Figure 1: Molecular phylogenies of subtilases ( a ) and vein patterning 1 (VEP1) ( b ). Numbers above branches show bootstrap values from maximum likelihood and distance analyses, respectively. Asterisks indicate values <50%. 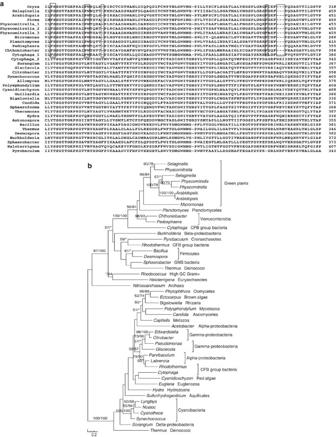Figure 2: Multiple sequence alignment (a) and molecular phylogeny (b) of acyl-activating enzymes 18 (AAE18). Boxed columns indicate the amino-acid residues and indels shared by bacterial and green plant AAE18 sequences. Numbers above branches show bootstrap values from maximum likelihood and distance analyses, respectively. Asterisks indicate values <50%. Full size image Figure 2: Multiple sequence alignment ( a ) and molecular phylogeny ( b ) of acyl-activating enzymes 18 (AAE18). Boxed columns indicate the amino-acid residues and indels shared by bacterial and green plant AAE18 sequences. Numbers above branches show bootstrap values from maximum likelihood and distance analyses, respectively. Asterisks indicate values <50%. Full size image Of the 57 gene families, 18 are present in both green algae and land plants, suggesting that they were likely acquired before the origin of land plants. The remaining 39 gene families are not found in green algae and might have been acquired during or after the origin of land plants. Notably, 19 of the identified gene families are only found in P. patens and their putative donors (prokaryotes, viruses or fungi) ( Table 1 ; Supplementary Table S1 ). All of these 19 families are located on large genomic scaffolds, indicating that they are unlikely to be bacterial contaminants. As P. patens is the only moss whose complete genome sequence is available, it is unclear whether these families also exist in other mosses or nonvascular land plants. However, the lack of homologues for these gene families in vascular plants suggests that they were likely transferred more recently to either P. patens or its close relatives. The vast majority of acquired gene families identified in our analyses are derived from miscellaneous bacterial lineages. Ten families are derived from fungi, and only one family is from archaea and viruses, respectively. As expected for land plants, which have often undergone frequent duplication events, 25 of identified gene families contain multiple copies in P. patens . In some cases, both acquired genes and endogenous homologues co-exist in P. patens . For instance, the gene family encoding FAD-linked oxidase comprises three identifiable copies in P. patens , two of which are closely related to CFB bacterial homologues and one may have been vertically inherited in eukaryotes ( Supplementary Fig. S1 ). A similar evolutionary scenario is also observed for the gene encoding phosphoenolpyruvate carboxylase (PEPCase). In this case, two PEPCase gene copies exist in P. patens , one of which is clearly related to proteobacterial sequences, whereas the other to those from photosynthetic eukaryotes, the chytrid fungus Spizellomyces , and other bacteria ( Supplementary Fig. S2 ). As HGT identification can be prone to errors owing to poor data quality and methodological limitations [19] , we have taken very cautious measures to alleviate these issues. These measures include construction of a comprehensive database, broad and balanced taxonomic sampling, careful inspection of alignments, determination of optimal protein substitution matrix for each data set and detection of other molecular characters consistent with the identified relationships. Such measures may have reduced most of the artifacts commonly encountered in HGT detection. It is critical to note that, although differential gene loss, sometimes associated with hidden paralogy, can always be invoked as an alternative explanation, HGT is the most parsimonious interpretation for the genes identified in Table 1 . This interpretation is consistent with independent evidence such as shared indels and amino-acid residues for many identified gene families ( Fig. 2 ; Supplementary Information ). On the other hand, the number of acquired genes in P. patens may have been underestimated in this study for several reasons. First, our study is primarily based on phylogenetic analysis, which, despite being considered the most reliable approach for HGT detection [35] , tends to have more false negatives owing to the lack of sufficient phylogenetic signal in many data sets. Second, only genes transferred from prokaryotes, viruses and fungi to plants were included in our results, those from other eukaryotes were not detected. Third, our results only include genes derived from a single HGT event (that is, genes transferred directly from their ultimate donors to mosses or to recent common ancestors of green plants). This might overlook genes involved in secondary or recurrent transfer events, which often lead to complex and patchy distributions [36] , [37] . Finally, our results are based solely on the analyses of the P. patens genome. Acquired genes in other land plants or secondarily lost in P. patens are not included. Therefore, our current results may only be viewed as a glimpse of acquired genes in land plants. HGT in plant development and adaptation Many of the genes identified in our analyses are related to essential or plant-specific metabolic and developmental processes (Table 1). Multiple gene families related to carbohydrate metabolism were acquired from bacteria, and they are involved in starch biosynthesis, cellulose degradation, pollen and seed germination as well as other activities in Arabidopsis . Another notable example is the large and versatile subtilase gene family. With subtilases of P. patens as queries, we were able to identify homologues only in bacteria and other land plants. Such sequence similarity is consistent with earlier reports that plant subtilases differ significantly from those of fungi and animals [38] . Further phylogenetic analyses indicate that land plant subtilases are derived from a single HGT event from bacteria, followed by rapid gene duplication ( Fig. 1a ). Our analyses also identified genes related to biosynthesis of plant polyamines and hormones. The gene encoding arginase is responsible for degrading arginine into ornithine, a major precursor for the biosynthesis of polyamines. Sequences of land plant arginase share 32–48% identities with those of bacterial agmatinase, but only 25–28% identities with arginase of other organisms. Consistent with the results of sequence comparisons, phylogenetic analyses indicate that land plant arginase evolved from bacterial agmatinase ( Supplementary Fig. S3 ). At least two acquired gene families, including those encoding acyl-activating enzyme 18 (AAE18) and YUCCA flavin monooxygenase (YUC3), are involved in the biosynthesis of auxin [39] , [40] , a hormone that regulates abscission suppression, apical dominance, cell elongation and xylem differentiation. Both AAE18 and YUC3 families were likely acquired from bacteria ( Fig. 2 ; Supplementary Fig. S4 ). In particular, plant AAE18 sequences share multiple conserved amino-acid residues and indels with homologues from planctomycetes, verrucomicrobia and CFB bacteria ( Fig. 2a ). Intriguingly, both the production and inhibition of auxin may be affected by the expression of acquired genes. In Arabidopsis , the bacteria-derived arginase (see above) may negatively regulate the production of auxin by reducing the level of nitric oxide, which in turn mediates the induction of auxin in roots [41] . Several other acquired gene families identified in our analyses are related to plant defence and stress tolerance ( Table 1 ). Notably, glutathione is essential for plant disease resistance, photo-oxidative stress defence and heavy metal detoxification [42] . Glutamate–cysteine ligase (GCL) is the first of the two enzymes catalysing the formation of glutathione. Identifiable homologues of P. patens GCL are only present in green plants and bacteria. Our phylogenetic analyses also show that the GCL gene was acquired from bacteria ( Supplementary Fig. S5 ), which is consistent with an earlier report [23] . In addition, at least three gene families acquired from bacteria, including guanine deaminase, allantoate amidohydrolase and ureidoglycolate amidohydrolase [43] , are involved in purine degradation and nitrogen recycling ( Table 1 ; Supplementary Figs S6 and S7 ). Furthermore, another acquired gene, glutamine synthetase, is directly responsible for assimilating ammonia into amino acids in plants ( Supplementary Fig. S8 ). Conventional belief is that HGT is frequent in unicellular eukaryotes but rare in multicellular eukaryotes because of the barriers of germline and apical meristem. Although evidence of HGT in multicellular eukaryotes is still limited, there have been numerous reports of acquired genes (including those of viral and bacterial origins) in mitochondrial genomes of seed plants [44] , [45] . These viral and bacterial genes were integrated into mitochondria and passed onto descendants ultimately through the apical meristem. Such observations, combined with other relatively recent HGT events reported in plants [13] , [17] and animals [16] , [18] , [46] , suggest that neither germline nor apical meristem constitutes an insurmountable barrier to HGT. The finding of 18 recently acquired gene families in mosses also raises questions why more foreign genes exist in this lineage and whether recent HGT of nuclear genes also occurs in other land plants. We reason that the acquisition of genes by mosses might largely be attributed to the unique evolutionary position and biological features of this lineage. As mosses were among the first dwellers on land, they might have encountered hostile environments with intense ultraviolet radiation [47] , which could break large DNA molecules into small fragments and release them into the environment. It is also known that mosses are effective in DNA transformation [48] . This ability to uptake foreign DNA, including beneficial genes from co-inhabitants, likely facilitated the establishment of these early land plants in a hostile and shifting environment. In addition, these early land plants formed mycorrhizal association with diverse fungal species [30] , [49] , and this symbiotic relationship provided further opportunities for gene transfer between fungi and early land plants [25] . Mosses also have distinct and dominant gametophytes in their lifecycle. As one of the earliest plant groups on land, mosses lack true vascular systems and complex protective structures for gametes and zygotes. We hypothesize that at least two entry points exist for foreign genes to be acquired and integrated into the moss nucleus ( Fig. 3 ). The first entry point for acquired genes is the stage of spore germination and early gametophyte development. Moss gametophytes are developed from haploid spores through mitosis. These gametophytes are simple, often relatively undifferentiated and prostrate in direct contact with soil surface, thus providing ample opportunities to uptake foreign DNA. In such cases, any genes acquired during spore germination and the early stage of gametophyte development could potentially be propagated into adult gametophytes, which bear either antheridia or archegonia or both. In the latter case, fertilization may also occur on the same gametophyte and lead to the fixation of acquired genes into zygotes and sporophytes. The second likely entry point for acquired genes in mosses is the stage of fertilization and early embryo development. Unlike seed plants where eggs are protected within ovules and fertilization entails a precise mechanism for pollen tube elongation and sperm delivery, mosses conceal eggs in single-layered and hollow archegonia, which are open during fertilization. Any foreign genes transferred from the exterior environment to exposed zygotes and young embryos will likely be fixed and passed onto adult sporophytes. 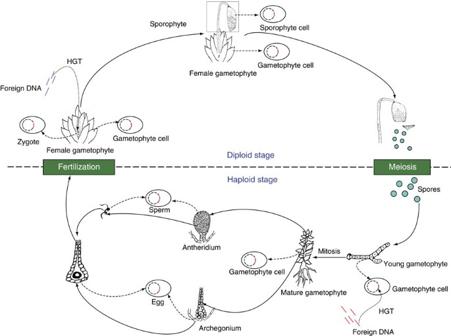Figure 3: A hypothetical scheme of HGT in mosses. Two entry points for foreign genes into the moss genome are proposed. The first entry point is spore germination and the early stage of gametophyte development. The second entry point is fertilization and the early stage of embryo development. This model is also applicable to other nonvascular plants and seedless vascular plants that have independent gametophytes. DNA acquired from foreign sources through the two entry points is shown in red and blue, respectively. Dash lines show the status of acquired genes in different stages of the lifecycle. Figure 3: A hypothetical scheme of HGT in mosses. Two entry points for foreign genes into the moss genome are proposed. The first entry point is spore germination and the early stage of gametophyte development. The second entry point is fertilization and the early stage of embryo development. This model is also applicable to other nonvascular plants and seedless vascular plants that have independent gametophytes. DNA acquired from foreign sources through the two entry points is shown in red and blue, respectively. Dash lines show the status of acquired genes in different stages of the lifecycle. Full size image The above model presumes that organisms with unprotected or weakly protected zygotes in their lifecycles are prone to HGT. This model predicts the existence of recently acquired genes in plants with independent, though sometimes reduced, gametophytes such as nonvascular and seedless vascular plants. Given the gradual transition of these early-branching land plants toward seed plants, this model also predicts the existence of anciently acquired genes in gymnosperms and angiosperms, where fertilization and embryogenesis are structurally internalized. It should be noted here that even such structural internalization might not entirely exclude recent HGT in gymnosperms and angiosperms. It is conceivable that pollen grains from distantly related plants may be deposited on the stigma of another plant, allowing foreign pollen DNA the chance to be transformed into the zygote and the young embryo [17] . The increasing structural complexity of land plants has been accompanied by diversified metabolic pathways and their chemical output. Like other complex multicellular eukaryotes, plants are able to form distinctive structures and coordinate development throughout their lifecycle. Our data clearly show that HGT contributed greatly to the metabolism, development and regulation of land plants. For example, members of the subtilase family participate in many biological processes, including protein degradation in seeds and fruits, lateral root formation, xylem differentiation, cuticle and epidermal development and stomata pattern formation [50] , [51] , [52] . Likewise, polyamines are involved in numerous important biological activities in plants such as translation, cell proliferation and signalling, ion channel regulation, and stress response [53] , [54] . Furthermore, plant hormones have a vital role in regulating cell differentiation and structural development. Land plants are also diverse in morphology, life history and habitat, and they have evolved many adaptive traits essential for their survival and development. Particularly during their transition from aquatic to terrestrial environments, plants evolved features to not only tolerate abiotic stress such as desiccation, fluctuating temperature and nutrient limitation, but also defend themselves against herbivory and microbial infection. Many of the acquired genes identified in our analyses are either directly or indirectly related to plant defence and stress tolerance. For instance, polyamines not only regulate calcium homeostasis and stomatal closure, but also are involved in plant tolerance to abiotic stress such as drought, salt and cold [53] . Given the role of arginase in polyamine biosynthesis, the acquisition of the arginase gene might benefit plants greatly as they adapt to water shortages, salinity and fluctuating temperatures on land. Similarly, the involvement of subtilases in the development of lateral roots, cuticle and stomatal cells also points to an important role of this gene family in water conduction as well as protection from desiccation and microbial infection in land plants. Additionally, several gene families identified in our analyses are functionally related to DNA replication and repair ( Table 1 ; Supplementary Figs S9, S10, S11 and S12 ). Given the fact that early land plants faced ubiquitous and intense ultraviolet radiation on earth surface [47] (which might cause DNA damage and consequently interrupt the normal cell cycle of plants), the acquisition of these genes may have conferred early land plants additional abilities to fix DNA damage and facilitate their survival. Such DNA repair-related genes have also been demonstrated to be of preferential uptake in some bacteria [55] . The cumulative impact of acquired genes depends critically on the number of such genes accumulated in a taxon. Genes acquired by any ancestral organism, if beneficial, are likely to be retained in descendent lineages. Indeed, 35 gene families identified in P. patens are also present in seed plants. Likewise, a considerable number of genes were transferred independently from bacteria during the early evolution of Plantae [31] , [32] . These data indicate that HGT is a dynamic process with foreign genes gradually accumulating over time ( Fig. 4 ). Such gradual accumulation of foreign genes in plants also suggests that anciently acquired genes are more frequent than commonly expected. 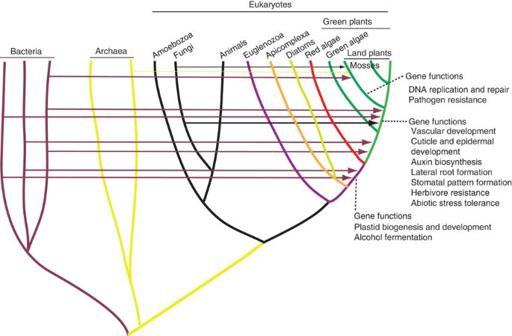Figure 4: Diagram illustrating the dynamics of HGT in plants. Horizontal lines and arrows show HGT donors and recipients. Information about HGT in the ancestor of red algae and green plants is based on31,32. Figure 4: Diagram illustrating the dynamics of HGT in plants. Horizontal lines and arrows show HGT donors and recipients. Information about HGT in the ancestor of red algae and green plants is based on [31] , [32] . Full size image Eukaryotic evolution has been significantly shaped by the origins of mitochondria and plastids, which routed numerous bacterial genes to the nucleus. Although such EGT events are often considered to be a dominant force in eukaryotic genome evolution, the sources of transferred genes are intrinsically constrained by the gene pool of mitochondria and plastids. With organellar genomes becoming increasingly reduced, the process of EGT will eventually approach to a dead end. The lack of such constraint for HGT, on the other hand, may potentially introduce genes of numerous sources and functions. The acquired genes identified in our analyses and their participation in diverse biological processes of land plants suggest a widespread and profound impact of HGT on the evolution of multicellular eukaryotes. Data sources and genome screening The annotated genome of P. patens was downloaded from the Joint Genome Institute. A customized database was created to search for P. patens gene homologues. In addition to NCBI non-redundant ( nr ) protein sequences, this customized database also included other sequenced genomes and expressed sequence tags from diverse eukaryotes ( Supplementary Table S2 ). Assembling of expressed sequence tag sequences was carried out using CAP3, and the resulting consensus sequences were translated using the OrfPredictor web server ( http://proteomics.ysu.edu/tools/OrfPredictor.html ). Genome screening for candidates of acquired genes was performed using a newly developed software package AlienG [34] with P. patens annotated protein sequences as query. AlienG presumes that sequence similarity is correlated to sequence relatedness. Therefore, if a query sequence is significantly more similar to homologues from distantly related organisms than to those from close relatives, it will be considered a candidate of acquired genes. Genes that are only detected in the query and potential donor groups (default E -value cutoff 1e-6) will also be identified. In this study, the significantly higher sequence similarity to homologues from a donor group was empirically set to a bit score ratio of over 1.5. All candidate genes identified by AlienG were subject to further sequence re-sampling and manual phylogenetic analyses to determine their evolutionary origins. Determining the origin for candidates of acquired genes For each candidate of acquired genes identified by AlienG, we first checked the scaffold on which the gene was located. Because of the potential contamination in the process of genome sequencing, any candidate of acquired genes located on a short scaffold was removed from further consideration. Detailed phylogenetic analyses, including sequence re-sampling from our internal customized sequence database, were performed for each of the remaining candidates. Taxonomic distribution of sequence homologues was also investigated. Because of the bacterial nature of mitochondria and plastids, we also investigated if other eukaryotic homologues were mitochondrial or plastid precursors, which often suggest a bacterial origin (see Supplementary Information ). Additionally, each alignment was carefully inspected for rare genomic characters that might indicate a close affinity between the candidate gene and homologues from the putative donor. A candidate gene was determined to be horizontally acquired based on (1) gene tree topology that shows a green plant/donor clade with bootstrap support of over 80% from maximum likelihood or distance analyses or both, (2) taxonomic distribution of homologues only in the putative donor group (bacteria, archaea, viruses or fungi) and (3) unique domain structures, indels or amino-acid residues shared with homologues from the putative donor group. Phylogenetic analyses Multiple protein sequence alignments were performed using MUSCLE and clustalX, followed by manual refinement. Gaps and ambiguously aligned sites were removed manually (alignments are available from the authors on request). Sequences that caused aberrant alignments and whose real identity could not be confirmed were also removed from alignments. Phylogenetic analyses were performed with a maximum likelihood method using PhyML 3.0 (ref. 56 ) and a distance method using neighbour of PHYLIPNEW v.3.68 (ref. 57 ) in EMBOSS package. ModelGenerator [58] was used to select the available model of protein substitution and rate heterogeneity that best fit each data set. Bootstrap support values were estimated using 100 pseudo-replicates. Maximum likelihood distances for distance analyses were calculated using TREE-PUZZLE v.5.2 (ref. 59 ) and PUZZLEBOOT v.1.03 (A. Roger and M. Holder, http://www.tree-puzzle.de ). The models used in maximum likelihood and distance analyses are the same in most cases. If the best model selected by ModelGenerator was not implemented in TREE-PUZZLE, the second best model was used. All other parameters in the analyses used default settings. Functional annotation Whenever possible, functional annotation of the acquired genes followed the information provided by The Arabidopsis Information Resources (TAIR) ( http://www.arabidopsis.org ) and published experimental data. Homologous gene loci in Arabidopsis were also obtained from TAIR. How to cite this article: Yue, J. et al . Widespread impact of horizontal gene transfer on plant colonization of land. Nat. Commun. 3:1152 doi: 10.1038/ncomms2148 (2012).